Ligand-engaged TCR is triggered by Lck not associated with CD8 coreceptor The earliest molecular events in T-cell recognition have not yet been fully described, and the initial T-cell receptor (TCR)-triggering mechanism remains a subject of controversy. Here, using total internal reflection/Forster resonance energy transfer microscopy, we observe a two-stage interaction between TCR, CD8 and major histocompatibility complex (MHC)-peptide. There is an early (within seconds) interaction between CD3ζ and the coreceptor CD8 that is independent of the binding of CD8 to MHC, but that requires CD8 association with Lck. Later (several minutes) CD3ζ–CD8 interactions require CD8–MHC binding. Lck can be found free or bound to the coreceptor. This work indicates that the initial TCR-triggering event is induced by free Lck. Antigen recognition by the T-cell receptor (TCR) is the first step in T-cell activation, and the paramount event for their development and functions. At the start of the signalling cascade, the immunoreceptor tyrosine-based activation motifs (ITAMs) of the CD3 signalling subunits of the TCR are phosphorylated by the Src-family kinase (SFK) Lck and, to a lesser extent, Fyn, and then bound by another kinase called ZAP70 (refs 1 , 2 , 3 ). After ZAP70 binds to CD3, the coreceptors CD4 or CD8, which are associated with the SFK Lck, become associated with the TCR–CD3 complex and bind to the major histocompatibility complex (MHC). This stabilizes the TCR-MHC-peptide (MHCp) interaction (at least in the case of CD8 (ref. 4 )), and Lck continues the phosphorylation of CD3 elements, ZAP70 and the many other downstream targets. Freshly isolated T cells, but not T cell lines, show partial phosphorylation of CD3ζ with bound but non-phosphorylated ZAP70 (ref. 5 ). This condition is thought to represent stimulation by self-MHCp in vivo [6] . Although TCR triggering has been extensively studied, the precise timing of signals downstream of the TCR is as yet poorly understood. TCR microclusters, in which signalling occurs, form at the immunological synapse (IS) within seconds of MHCp recognition [7] . Using MHC complexes containing an antigenic peptide that is biologically inert until exposed to ultraviolet light, Huse et al. [8] developed a high-resolution temporal analysis of signalling. Phosphorylation of the adaptor molecule linker for activation of T cells (LAT) was observed within 4 s, and diacylglycerol production and calcium flux was observed after 6–7 s (ref. 8 ). A recent biophysical study on TCR and CD8 binding to MHCp demonstrated that the initial binding of TCR to MHCp induces, in a SFK-dependent manner, the binding of CD8 to the MHCp [9] , leading to the question of how the TCR–CD3 complex is initially phosphorylated by an SFK before CD8 and the associated Lck have been recruited to the TCR–CD3 complex. CD8 coreceptor is expressed on cytotoxic T lymphocytes and their double-positive thymic progenitors, where its main function is to augment the sensitivity and response of T cells to cognate MHCp ligands [4] , [10] . It is generally accepted that the ability of the coreceptor to enhance T-cell responses is due to two main effects: (i) Binding of CD8 to MHC class I (MHCI) molecules helps stabilize weak TCR–MHCp interactions; (ii) the recruitment of Lck, which is bound to the cytoplasmic tail of the coreceptor, to the TCR complex upon coreceptor binding to the MHC, thereby enhancing the initiation of TCR signalling [4] , [11] . Lck consists of N-terminal sequences that mediate its myristoylation, palmitoylation and association with coreceptors, followed by SH3, SH2 and tyrosine kinase domains, and C-terminal negative regulatory domain [12] . Lck can be found either free in the cytosol [13] , anchored to the plasma membrane through myristoylation and palmitoylation, or associated with the CD8 or CD4 coreceptors through a ‘zinc-clasp’ structure [14] . Lck activity is largely controlled by the equilibrium between phosphorylation and dephosphorylation at a C-terminal inhibitory tyrosine (Y 505 ) and an activating tyrosine in the catalytic domain (Y 394 ) [2] . Relatively high amounts (up to ~40%) of constitutively active pY 394 -Lck are present in resting T cells and thymocytes [15] , suggesting an important role of spatial organization of Lck and TCR in regulation of TCR triggering [16] . Lck also has a poorly understood kinase-independent function [17] . Chimeric proteins formed by CD4 fused to Lck with a deleted kinase domain were shown to be more efficient at supporting full activation of a CD4-dependent T-cell hybridoma than the full-length chimeric fusion protein [18] . This kinase-independent activity was largely dependent on intact SH2, SH3 domains as well as presence of intact endogenous Lck in the CD4-deficient T-cell hybridoma [19] . Importantly, CD8α-Lck kinase-dead fusion protein could reconstitute thymic development in MHCI-restricted TCR transgenic CD8α-deficient mice [20] , suggesting that one of the functions of Lck is to serve as an adaptor molecule that regulates the interactions of the coreceptor with MHC and TCR [18] . Previously, we used Forster resonance energy transfer (FRET) microscopy in live and fixed cells to investigate the interaction of CD4 or CD8 with TCR, using CD3ζ-cyan fluorescent protein (CFP) as FRET donor and CD4-yellow fluorescent protein (YFP) or CD8β-YFP as FRET acceptors [21] , [22] , [23] , [24] . We showed that the coreceptors interact with the TCR only after recognition of antigenic MHCp, but CD8 can be recruited to the IS independently of the sequence of peptide presented on MHC [21] , [22] , [23] . We also found that the strength of the interaction measured by FRET between the TCR complex and CD8 corresponded closely to the strength of T-cell activation by particular peptides, and that differences in FRET kinetics during recognition of different MHCp ligands correlated closely to the ability of a particular ligand to induce positive or negative selection in thymocytes [24] , [25] . However, the temporal resolution of these studies was limited, and they could not provide more detailed information about the sequence of molecular events during TCR triggering. We therefore decided to look more closely at the earliest stages of the interaction using the higher-spatial and temporal resolution afforded by total internal reflection (TIRF) microscopy of T cells interacting with supported lipid bilayers as model antigen-presenting surfaces [26] . In the present study, we show conclusively that TCR triggering occurs in two distinct stages: early phosphorylation of TCR–CD3 by Lck that is not associated with the coreceptor leading to MHC-independent association between CD8 and TCR–CD3, followed later by MHC-dependent CD3–CD8 interaction [3] , [9] , [17] . The free, active Lck initiates TCR–CD3 complex phosphorylation, whereas the coreceptor-associated Lck acts mainly as an adaptor molecule, recruiting CD8 to the phosphorylated TCR–CD3 complex through direct binding to phospho-CD3 or to phospho-ZAP70 associated with phosphorylated CD3. Antigen induced CD8β–CD3ζ interaction We first assessed the relationship between CD8 recruitment to the immune synapse and its ability to bind to MHCp by analysing the synapses formed between OT-I T-cell hybridomas expressing CD3ζ-CFP and CD8α,β-YFP (hybridoma cell line hence referred to as OT-I.ZC.8βY) cells [23] , and a surrogate antigen-presenting cell line: CHO cells expressing either inducible wild-type scH-2K b -OVA or a D 227 K/E 229 K mutant that cannot bind to CD8 (scH2-K b -OVA-CD8 mut ). These sc-MHCI constructs were described previously [27] . The OT-I TCR recognizes the agonist OVA peptide (SIINFEKL) with high affinity, but not the VSV peptide (RGYVYQGL), when either is presented by H-2K b . We compared the intensity of CD8β-YFP fluorescence in the immune synapse, showing that the CD8 recruitment itself was not solely a result of TCR recognition of MHCp, but instead was driven by the CD8–MHCI interaction ( Fig. 1a ), as indicated by our earlier work [23] , [28] . 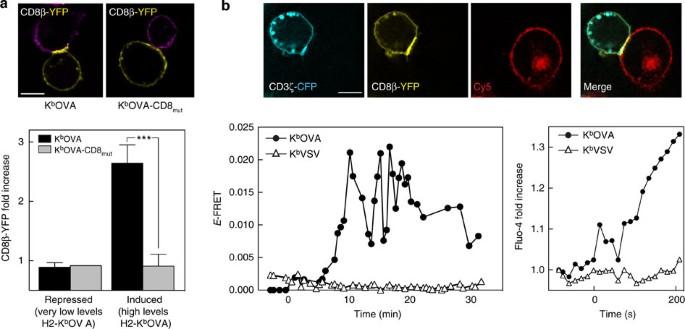Figure 1: Recruitment of CD8 and imaging of the induction of TCR–CD8 FRET by an agonist. (a) OT-I hybridomas expressing CD8α wild-type, CD3ζ-CFP and CD8β-YFP (OT-I.ZC.8βY) were incubated with Cy5-stained CHO cells expressing tetracycline-induced wild-type single-chain H2-KbOVA (left) or a mutant that cannot bind to CD8 (right). The image of each panel shows mid-cell sections of fluorescence images (CD8β-YFP in yellow and Cy5 in purple). Scale bar, 5 μm. The bottom graph shows the quantitation of CD8β-YFP recruitment to the immune synapse when scH2-Kb-OVA (black) or scH2-Kb-CD8mut-OVA (grey) was expressed on CHO cells’ surface. Mean fluorescence intensity ±s.e.m.,n=25 conjugates. Unpairedt-test; *P<0.0001. (b) Top row shows a representative image of OT-I.ZC.8βY cells forming the immune synapse formation (CD3ζ-CFP in cyan, CD8β-YFP in yellow and CHO APC membrane labelled with Cy3.5 in red). Bottom-left plot shows live FRET efficiency of OT-I.ZC.8βY cells incubated with scH2-Kb-OVA (closed circles) or -VSV (open triangles) expressing CHO cells. Data represent average FRET efficiency at the synapse. Bottom-right panel shows Ca2+flux from a Fluo-4-loaded OT-I cell expressing CD8α/CD8β during interaction with a CHO cell expressing scH2-Kb-OVA (circles) or -VSV (triangles). The results are representative of at least three independent experiments. Figure 1: Recruitment of CD8 and imaging of the induction of TCR–CD8 FRET by an agonist. ( a ) OT-I hybridomas expressing CD8α wild-type, CD3ζ-CFP and CD8β-YFP (OT-I.ZC.8βY) were incubated with Cy5-stained CHO cells expressing tetracycline-induced wild-type single-chain H2-K b OVA (left) or a mutant that cannot bind to CD8 (right). The image of each panel shows mid-cell sections of fluorescence images (CD8β-YFP in yellow and Cy5 in purple). Scale bar, 5 μm. The bottom graph shows the quantitation of CD8β-YFP recruitment to the immune synapse when scH2-K b -OVA (black) or scH2-K b -CD8 mut -OVA (grey) was expressed on CHO cells’ surface. Mean fluorescence intensity ±s.e.m., n =25 conjugates. Unpaired t -test; * P <0.0001. ( b ) Top row shows a representative image of OT-I.ZC.8βY cells forming the immune synapse formation (CD3ζ-CFP in cyan, CD8β-YFP in yellow and CHO APC membrane labelled with Cy3.5 in red). Bottom-left plot shows live FRET efficiency of OT-I.ZC.8βY cells incubated with scH2-K b -OVA (closed circles) or -VSV (open triangles) expressing CHO cells. Data represent average FRET efficiency at the synapse. Bottom-right panel shows Ca 2+ flux from a Fluo-4-loaded OT-I cell expressing CD8α/CD8β during interaction with a CHO cell expressing scH2-K b -OVA (circles) or -VSV (triangles). The results are representative of at least three independent experiments. Full size image Because of the differences in timing between our previous measurements of FRET between TCR and coreceptors [21] , [23] , [24] , and other’s analyses of early signalling events during T-cell antigen recognition [8] , [9] , we decided to further characterize the TCR–CD8 interaction. The interaction between two molecules can be studied using FRET, which occurs only between molecules separated by 10 nm or less. After donor excitation, FRET leads, due to the energy transfer, to decreased donor fluorescence and increased acceptor fluorescence [29] . We allowed CHO cells expressing either sc-H-2K b -OVA or sc-H-2K b -VSV to settle in a 37-°C-heated chamber before the addition of OT-I.ZC.8βY cells. We monitored the interaction between CD3ζ-CFP and CD8β-YFP by live FRET efficiency (E-FRET) imaging during the process of antigen recognition [21] , [30] . After stimulation with sc-H-2K b -OVA-expressing cells, both CD3ζ-CFP and CD8β-YFP were recruited to the synapse, where the FRET signal between CD3ζ-CFP and CD8β-YFP began to increase strongly about 5 min after the beginning of the antigen-presenting cell (APC)–T-cell interaction ( Fig. 1b ) until it peaked at 10 min, remaining oscillating for another 10 min and then decreasing. No detectable FRET was found at any time when the T cells interacted with the non-stimulatory sc-H-2K b -VSV-expressing CHO cells. These results agreed with previous studies from this lab [23] , [24] , but we considered it likely that we were underestimating the timing and the potency of the interaction owing to technical limitations of the experimental setup, and to the fact that we were analysing the average FRET efficiency over the whole synapse. During the interaction of sc-H-2K b -OVA-expressing CHO cells with 17αβ cells (T-cell hybridoma expressing OT-I TCR and CD8αβ) loaded with the Ca 2+ fluorescent indicator Fluo-4, cytosolic Ca 2+ concentration [Ca 2+ ] i increased at the very moment that the initiation of the interaction was observed ( Fig. 1b , right plot). This suggested that we were indeed missing early signalling events. Looking closely at the FRET data in Fig. 1b , we noted that there appeared to be a slight rise in the E-FRET signal at the time of contact between the T cell and the APC, which continued until the main E-FRET increase at ~5 min. While its significance was questionable, we hypothesized that this could represent small localized regions of TCR–CD8 interaction that were ‘diluted’ in the analysis of the whole synapse. To improve the resolution of our imaging, we used artificial supported lipid bilayers as antigen-presenting surfaces [26] , [31] , imaging the IS between the T cell and the bilayer presenting H-2K b –peptide complex as well as ICAM-1 ( Fig. 2a ). We used a TIRF microscopy system that allowed us to increase spatial resolution by exciting only the fluorophores immediately adjacent to the glass–oil interface ( z =100 nm), in other words, imaging the immune synapse. The bilayers were fully functional as surrogate antigen-presenting surfaces, supporting full lipid motility, determined by fluorescence recovery after photobleaching ( Supplementary Fig. 1a ) and antigen-specific T-cell activation (determined by MHCp relocation in Supplementary Fig. 1b , Ca 2+ flux in Supplementary Fig. 1c and total phosposhotyrosine imaging in Supplementary Fig. 1d ). We switched fluorophores to green and red fluorescent proteins (enhanced green fluorescent protein (eGFP) as donor and mCherry as acceptor) to be compatible with the TIRFM system. Thus, using a new hybridoma cell line expressing CD3ζ-eGFP and CD8β-mCherry, hence referred to as OT-I.ZG.8βR, T cells stimulated by H-2K b -OVA bilayers we were able, not only to reproduce the kinetics of our previous results in live and fixed cells, but also to detect a weak but significant increase in FRET efficiency in the earliest time point analysed (1 min) ( Fig. 2b,c ). This FRET signal was not observed in T cells interacting with bilayers presenting the non-stimulatory H-2K b –VSV complexes. This early FRET was observed in small localized clusters. This likely corresponds to the very early moments of antigen recognition, taking into account that it takes about 30–60 s for the settling cells to reach the bilayer. After this initial CD3ζ–CD8β interaction, a stronger interaction occurred after about 5 min. These results clearly indicate a two-stage interaction process. 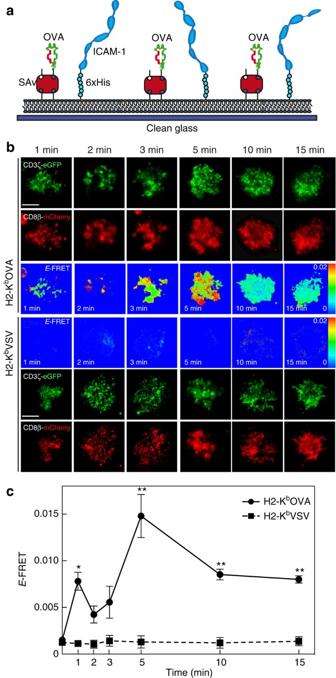Figure 2: Induction of TCR–CD8 FRET by an agonist on artificial lipid bilayers. (a) Scheme of supported lipid bilayers used as artificial antigen presenting surfaces. (b) OT-I hybridomas expressing CD8α wild-type, CD3ζ-eGFP and CD8β-mCherry (OT-I.ZG.8βR) were added to lipid bilayers containing either H2-Kb-OVA or H2-Kb-VSV monomers and ICAM-1, fixed at the indicated time points and imaged by TIRFM at the immune synapses. Images shown in green represent CD3ζ-eGFP, CD8β-mCherry in red and FRET efficiency in false colour scale. Images are representative of three different experiments. Scale bar, 5 μm. (c) FRET efficiency analysis of immune synapses from OT-I.ZG.8βR interacting with lipid bilayers containing H2-Kb-OVA (circles). Mean±s.e.m. of 1 minn=18, 2 minn=33, 3 minn=18, 5 minn=45, 10 minn=50 and 15 minn=52. Or H2-Kb-VSV bilayers (squares), mean±s.e.m. of 1 minn=12, 2 minn=15, 3 minn=13, 5 minn=21, 10 minn=14 and 15 minn=13. Unpairedt-test. *P<0.01 and **P<0.001. Figure 2: Induction of TCR–CD8 FRET by an agonist on artificial lipid bilayers. ( a ) Scheme of supported lipid bilayers used as artificial antigen presenting surfaces. ( b ) OT-I hybridomas expressing CD8α wild-type, CD3ζ-eGFP and CD8β-mCherry (OT-I.ZG.8βR) were added to lipid bilayers containing either H2-K b -OVA or H2-K b -VSV monomers and ICAM-1, fixed at the indicated time points and imaged by TIRFM at the immune synapses. Images shown in green represent CD3ζ-eGFP, CD8β-mCherry in red and FRET efficiency in false colour scale. Images are representative of three different experiments. Scale bar, 5 μm. ( c ) FRET efficiency analysis of immune synapses from OT-I.ZG.8βR interacting with lipid bilayers containing H2-K b -OVA (circles). Mean±s.e.m. of 1 min n =18, 2 min n =33, 3 min n =18, 5 min n =45, 10 min n =50 and 15 min n =52. Or H2-K b -VSV bilayers (squares), mean±s.e.m. of 1 min n =12, 2 min n =15, 3 min n =13, 5 min n =21, 10 min n =14 and 15 min n =13. Unpaired t -test. * P <0.01 and ** P <0.001. Full size image CD8β–CD3ζ interaction is a two-stage process A recent study also suggests biphasic TCR and CD8 interactions with peptides presented by MHCI [9] . In the first step, TCR binds MHCp, causing SFK activity that is a pre-requisite for the second stage, when CD8 binds MHCI [9] . The CD8–MHCI interaction stabilizes the interaction between the three molecules. Thus the kinase activity of the first stage occurs before CD8 has had a chance to associate with the MHCI. Since the SFK Lck is thought to be associated with the coreceptor, the mechanism for the initial phosphorylation step is unclear [3] . Using a T-cell hybridoma expressing OT-I TCR with CD3ζ-eGFP, CD8α and a S 101 A/K 103 D CD8β mutant that cannot bind to MHCI, CD8β-MHC mut -mCherry (hence referred to as OT-I.ZG.8β-MHC mut R) [23] , [28] , [32] . We observed an early CD3–CD8 FRET signal in T cells expressing the CD8 mutant that cannot bind to MHC, when exposed to MHCp complexes, and this FRET signal was comparable to the signal observed for T cells expressing wild-type CD8 ( Fig. 3a ). In contrast, CD8 unable to bind MHCI did not interact with CD3 at 15 min, and did not enable T-cell activation ( Fig. 3a,b ). To further confirm the importance of CD8 binding to MHCI for the late FRET signals, we tested the activation state of the cells (15 min) by total phospho-Tyr staining and compared total phospho-Tyr levels in cells expressing wild-type CD8 in response to wild-type MHCI monomers or with chimeric monomers consisting of mouse α1α2 heavy chain and human α3 domain that cannot bind to mouse CD8 (H-2K b -OVA-HLA-A*02:01) [9] presented on the bilayers with cells expressing CD8 mutant that cannot bind MHCI ( Fig. 3c ). In addition, we used primary OT-I cytotoxic T lymphocyte (CTL) cells plus or minus CD8-blocking antibodies in bilayers presenting wild-type MHCI molecules or MHCI molecules that cannot bind CD8 ( Fig. 3d ). When the blocking anti-CD8 antibody (Ab) was present, or in response to MHCI mutant, total phospho-Tyr activity was as low as when the non-stimulatory VSV peptide was presented ( Fig. 3c,d ). 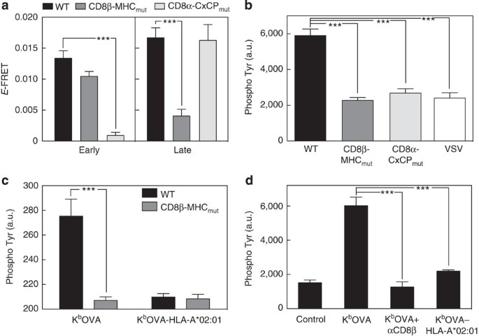Figure 3: Two-stage interaction between TCR and CD8. (a) OT-I hybridomas expressing CD8αWT, CD3ζ-eGFP and CD8β-mCherry (black); CD8αWT, CD3ζ-eGFP and CD8β-MHCmut-mCherry (dark grey) or CD8α-CxCPmut, CD3ζ-eGFP and CD8β-mCherry (light grey) were added to lipid bilayers containing Kb-OVA and ICAM-1, fixed at 1 min (‘early’) or 10 min (‘late’), and imaged by TIRFM at the immune synapses. FRET efficiency ±s.e.m. was plotted, ‘early’ WT (n=30), CxCPmut(n=25), MHCmut(n=28), and ‘late’n=28, 24, 29, respectively. (b) OT-I hybridomas expressing CD8αβ WT (black), CD8αβ-MHCmut(dark grey) or CD8α-CxCPmutand CD8β WT (light grey) were stimulated as inafor 15 min and stained with anti-phospho-Tyr. Images were taken using TIRFM. Mean fluorescence of WTn=20, MHCmutn=33, CxCPmutn=36 and VSVn=21±s.e.m. is shown. OT-I cells expressing CD8αβ-WT (white) were added to bilayers containing Kb-VSV and ICAM-1 as a negative control. (c) OT-I hybridomas expressing CD8αβ-WT (black) or CD8αβ-MHCmut(dark grey) were added to bilayers containing either Kb-OVA or Kb-OVA-HLA-A*02:01 plus ICAM-1 for 15 min, then stained with anti-phospho-Tyr. Mean fluorescence ±s.e.m. shown for Kb-OVA, WTn=15; CD8β-MHCmutn=15 and for Kb-OVA-HLA-A*02:01 WTn=15; CD8β-MHCmutn=19. (d) Primary mouse OT-I CTL were pretreated with blocking anti-CD8 (dark grey) or directly (black) added to bilayers containing either Kb-OVA or Kb-OVA-HLA-A*02:01 plus ICAM-1 or ICAM-1 alone (control) for 15 min, then stained with anti-phospho-Tyr. Mean fluorescence of controln=23, Kb-OVAn=17, anti-CD8βn=19 and Kb-OVA-HLA-A*02:01n=20±s.e.m. are shown. Unpairedt-test. ***P<0.0001. Figure 3: Two-stage interaction between TCR and CD8. ( a ) OT-I hybridomas expressing CD8αWT, CD3ζ-eGFP and CD8β-mCherry (black); CD8αWT, CD3ζ-eGFP and CD8β-MHC mut -mCherry (dark grey) or CD8α-CxCP mut , CD3ζ-eGFP and CD8β-mCherry (light grey) were added to lipid bilayers containing K b -OVA and ICAM-1, fixed at 1 min (‘early’) or 10 min (‘late’), and imaged by TIRFM at the immune synapses. FRET efficiency ±s.e.m. was plotted, ‘early’ WT ( n =30), CxCP mut ( n =25), MHC mut ( n =28), and ‘late’ n =28, 24, 29, respectively. ( b ) OT-I hybridomas expressing CD8αβ WT (black), CD8αβ-MHC mut (dark grey) or CD8α-CxCP mut and CD8β WT (light grey) were stimulated as in a for 15 min and stained with anti-phospho-Tyr. Images were taken using TIRFM. Mean fluorescence of WT n =20, MHC mut n =33, CxCP mut n =36 and VSV n =21±s.e.m. is shown. OT-I cells expressing CD8αβ-WT (white) were added to bilayers containing K b -VSV and ICAM-1 as a negative control. ( c ) OT-I hybridomas expressing CD8αβ-WT (black) or CD8αβ-MHC mut (dark grey) were added to bilayers containing either K b -OVA or K b -OVA-HLA-A*02:01 plus ICAM-1 for 15 min, then stained with anti-phospho-Tyr. Mean fluorescence ±s.e.m. shown for K b -OVA, WT n =15; CD8β-MHC mut n =15 and for K b -OVA-HLA-A*02:01 WT n =15; CD8β-MHC mut n =19. ( d ) Primary mouse OT-I CTL were pretreated with blocking anti-CD8 (dark grey) or directly (black) added to bilayers containing either K b -OVA or K b -OVA-HLA-A*02:01 plus ICAM-1 or ICAM-1 alone (control) for 15 min, then stained with anti-phospho-Tyr. Mean fluorescence of control n =23, K b -OVA n =17, anti-CD8β n =19 and K b -OVA-HLA-A*02:01 n =20±s.e.m. are shown. Unpaired t -test. *** P <0.0001. Full size image Lck-CD8 interaction is required for initial CD8 recruitment To test whether CD8 needed to be bound to Lck to interact with the TCR–CD3 complex after antigen recognition, we imaged early and late FRET signals during antigen recognition by OT-I T-hybridoma cells expressing CD3ζ-eGFP, CD8β-mCherry and CD8 with a mutation of the intracellular CxCP motif that mediates the interaction with Lck (hence referred to as OT-I.ZG.8αCxCP mut /8β.R). The C 227 KC 229 P motif was mutated to S 227 KS 229 P (ref. 33 ). This experiment showed that the Lck-binding mutation completely abrogated the early interaction between CD3ζ-GFP CD8β-mCherry as well as the later phospho-Tyr signalling ( Fig. 3a,b ). This suggests that the Lck interaction with CD8 was required to bring CD8 close to the TCR–CD3 complex at an early time point. The interaction between MHCI and CD8 is strong enough to overcome this effect at later time points, as indicated by the recovery of the second interaction stage ( Fig. 3a ). CD8–Lck and MHCp interactions required for two-stage kinetics Our FRET data strongly suggest that CD8 interactions with TCR–CD3 occur in two stages, with the early (<1 min) stage requiring CD8 binding to Lck, but not to MHC, and the late (>5 min) stage requiring CD8 binding to MHC, but not to Lck. We validated the relevance of this finding using the adhesion frequency assay for analysis of two-dimensional binding described previously [9] , [34] , [35] . In brief, an OT-I T-hybridoma cell with various combinations of transduced signalling proteins and a red blood cell (RBC) bearing H-2K b -OVA were aspirated by respective pipettes and driven in and out of contact with controlled area and duration. Adhesion was defined as stretching of the RBC on T-cell retraction [9] . This contact–retraction cycle was repeated 50 times for a given contact duration on each cell pair. We performed two-dimensional binding studies with the three different hybridomas expressing either wild-type CD8 molecules, or CD8 with abrogated binding to Lck or MHC. The kinetics of their interactions with K b -OVA, were expressed as the normalized adhesion bonds <n>/m pMHC . Plots of <n>/m pMHC of cells expressing OT-I TCR with CD3ζ, CD8α and CD8β showed two-stage kinetics, whereas plots from cells expressing either CD8α-CxCP mut ( Fig. 4a ) or CD8β-MHC mut ( Fig. 4b ) showed single-stage kinetics. This confirmed that the Lck interaction with CD8 was required to bring CD8 close to the TCR, and that the CD8–MHCI interaction was responsible for the second binding stage that results in the late FRET peak. 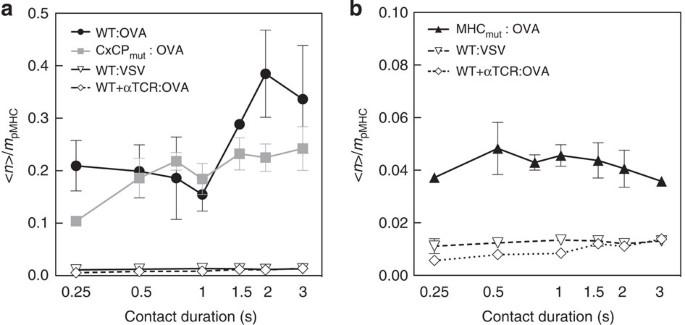Figure 4: Adhesion frequency assay. (a) Frequency of adhesion was normalized to the amount of pMHC presented (<n>/mpMHC) and plotted against timetfor OT-I hybridomas expressing CD8α wild-type and CD8β-wild-type (closed circles), or CD8α-CxCPmutand CD8β wild-type (closed squares) T cells interacting with RBCs bearing 4 and 7 OVA:H-2Kbper mm2, respectively, at 37 °C. Controls with CD8 wild-type cells pretreated with a blocking antibody against TCR (open diamond), or using RBCs bearing 93 VSV:H-2Kbper mm2(open triangle) were conducted. Representative data from three repeated experiments are shown. (b)<n>/mpMHCversustdata of OT-I hybridomas expressing CD8α wild-type and CD8β-MHCmut(closed triangles) T cells interacting with RBCs bearing 23 OVA:H-2Kbper μm2. Controls with CD8 wild-type cells pretreated with a blocking antibody against TCR (open diamond), or using RBCs bearing 93 VSV:H-2Kbper mm2(open triangle) were conducted. Data are representative of three experiments. Figure 4: Adhesion frequency assay. ( a ) Frequency of adhesion was normalized to the amount of pMHC presented ( <n>/m pMHC ) and plotted against time t for OT-I hybridomas expressing CD8α wild-type and CD8β-wild-type (closed circles), or CD8α-CxCP mut and CD8β wild-type (closed squares) T cells interacting with RBCs bearing 4 and 7 OVA:H-2K b per mm 2 , respectively, at 37 °C. Controls with CD8 wild-type cells pretreated with a blocking antibody against TCR (open diamond), or using RBCs bearing 93 VSV:H-2K b per mm 2 (open triangle) were conducted. Representative data from three repeated experiments are shown. ( b ) <n>/m pMHC versus t data of OT-I hybridomas expressing CD8α wild-type and CD8β-MHC mut (closed triangles) T cells interacting with RBCs bearing 23 OVA:H-2K b per μm 2 . Controls with CD8 wild-type cells pretreated with a blocking antibody against TCR (open diamond), or using RBCs bearing 93 VSV:H-2K b per mm 2 (open triangle) were conducted. Data are representative of three experiments. Full size image To investigate TCR triggering in primary T cells, CTLs were prepared from OT-I TCR transgenic mouse splenocytes after activation by OVA peptide with addition of interleukin (IL)-2. CTLs were transduced with a biosensor for CD3 ITAM phosphorylation consisting of mCherry fused to the tandem SH2 domains of ZAP70 (mCherry-tSH2(ZAP70)) [36] . In resting T cells ZAP70 is located in the cytosol, but upon TCR activation it relocates to the plasma membrane through association of its SH2 domains to the phosphorylated ITAMs of the CD3 complex. This translocation can be detected by fluorescence microscopy upon T-cell activation after crosslinking with anti-CD3+anti-CD8 ( Fig. 5a ). Due to the optical characteristics of TIRF illumination, this sensor is extremely useful to analyse T-cell activation at the immune synapse. After adding OT-I CTL expressing the mCherry-tSH2(ZAP70) biosensor to lipid bilayers presenting specific MHCp (H-2K b -OVA), we observed consistent presence of mCherry-tSH2(ZAP70), indicating CD3 ITAM phosphorylation, in the immune synapse. With bilayers presenting the chimeric variant that cannot bind to CD8 (H-2K b -OVA-HLA-A*02:01), early but transient accumulations of ZAP70 were noted ( Fig. 5b ). 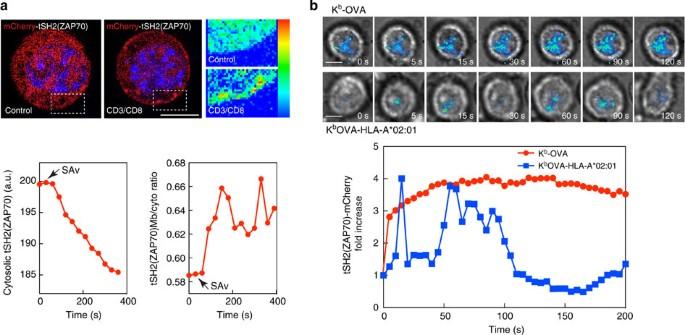Figure 5: CD8/MHCp interaction is required for sustained signaling through the TCR. (a) Nuclei of OT-I primary CTL expressing mCherry-tSH2(ZAP70) were stained with the live cell-imaging-compatible Hoechst 33342 and then incubated with a mixture of biotinylated anti-CD3ε and anti-CD8β antibodies and imaged under a deconvolution microscope. Top row shows the localization of mCherry-tSH2(ZAP70) before (left) and after the addition of crosslinking streptavidin (right). Higher detail in zoomed boxes in false colour. Bottom, graphs showing decrease in cytosolic fluorescence after streptavidin addition (left) in selected regions, or ratio between membrane and cytosolic fluorescence (right). Data are representative of at least three different experiments. Scale bar, 5 μm. (b) OT-I primary CTL cells expressing mCherry-tSH2(ZAP70) were added to lipid bilayers containing either H2-Kb-OVA or H2-Kb-OVA-HLA-A*02:01 monomers and ICAM-1, and analysed by live cell TIRFM at the immune synapses. Representative time points are shown in the top rows where the cells can be seen by transmitted light and the recruitment of mCherry-tSH2(ZAP70) is shown as a false colour overlayed image. Bottom graph, normalized mean mCherry-tSH2(ZAP70) fluorescence at the immune synapse in bilayers containing either H2-Kb-OVA (red) or H2-Kb-OVA-HLA-A*02:01 (blue). Data are representative of three experiments. Figure 5: CD8/MHCp interaction is required for sustained signaling through the TCR. ( a ) Nuclei of OT-I primary CTL expressing mCherry-tSH2(ZAP70) were stained with the live cell-imaging-compatible Hoechst 33342 and then incubated with a mixture of biotinylated anti-CD3ε and anti-CD8β antibodies and imaged under a deconvolution microscope. Top row shows the localization of mCherry-tSH2(ZAP70) before (left) and after the addition of crosslinking streptavidin (right). Higher detail in zoomed boxes in false colour. Bottom, graphs showing decrease in cytosolic fluorescence after streptavidin addition (left) in selected regions, or ratio between membrane and cytosolic fluorescence (right). Data are representative of at least three different experiments. Scale bar, 5 μm. ( b ) OT-I primary CTL cells expressing mCherry-tSH2(ZAP70) were added to lipid bilayers containing either H2-K b -OVA or H2-K b -OVA-HLA-A*02:01 monomers and ICAM-1, and analysed by live cell TIRFM at the immune synapses. Representative time points are shown in the top rows where the cells can be seen by transmitted light and the recruitment of mCherry-tSH2(ZAP70) is shown as a false colour overlayed image. Bottom graph, normalized mean mCherry-tSH2(ZAP70) fluorescence at the immune synapse in bilayers containing either H2-K b -OVA (red) or H2-K b -OVA-HLA-A*02:01 (blue). Data are representative of three experiments. Full size image When primary OT-I CTLs were analysed by western blot for specific phosphorylation of CD3ζ and for Ca 2+ flux, after stimulation with H-2K b -OVA tetramer, we confirmed that the initial CD3ζ phosphorylation and Ca 2+ transients were high and sustained ( Fig. 6 ). When the tetramers were unable to bind to CD8 there was only a small initial peak of CD3ζ phosphorylation, and a Ca 2+ flux that was not sustained over time. CD3ζ phosphorylation was completely inhibited by addition of the SFK inhibitor PP2 ( Fig. 6 ; Supplementary Fig. 3a ). Together these data confirm, as expected, the importance of CD8–MHCI interaction for the stabilization of the trimolecular complex and for maintenance of the TCR signalling process. More interestingly, these data also demonstrate an initial SFK-dependent phosphorylation of ITAMs on the CD3 complex that is independent of the coreceptor binding to MHC. 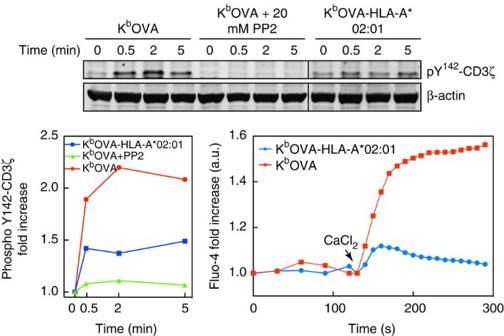Figure 6: Src kinase family activity is responsible of TCR phosphorylation after antigen recognition. Primary OT-I CTL were pretreated or not with the general Src kinase inhibitor PP2 (20 mM) and then stimulated with either H2-Kb-OVA or H2-Kb-OVA-HLA-A*02:01 tetramers for the indicated times. CD3ζ phosphorylation was analysed by immunoblot. Quantification of band intensities is shown in the left plot. In the right-hand plot, cells were loaded with Ca2+-sensitive dye Fluo-4 and imaged after the addition on top of bilayers containing either H2-Kb-OVA or H2-Kb-OVA-HLA-A*02:01 monomers plus ICAM-1, as described in the Methods section. Data are representative of four experiments. Data are representative of three experiments. Figure 6: Src kinase family activity is responsible of TCR phosphorylation after antigen recognition. Primary OT-I CTL were pretreated or not with the general Src kinase inhibitor PP2 (20 mM) and then stimulated with either H2-K b -OVA or H2-K b -OVA-HLA-A*02:01 tetramers for the indicated times. CD3ζ phosphorylation was analysed by immunoblot. Quantification of band intensities is shown in the left plot. In the right-hand plot, cells were loaded with Ca 2+ -sensitive dye Fluo-4 and imaged after the addition on top of bilayers containing either H2-K b -OVA or H2-K b -OVA-HLA-A*02:01 monomers plus ICAM-1, as described in the Methods section. Data are representative of four experiments. Data are representative of three experiments. Full size image A small amount of Lck is enough to phosphorylate the TCR Several lines of evidence indicate that the initial phosphorylation of CD3ζ ITAMs and ZAP70 is mediated by Lck and/or Fyn [37] , [38] , [39] . Lck-deficient mice have stronger defects in most aspects of signalling than Fyn-deficient mice [40] , yet the mechanism of the process that initiates the TCR signalling cascade is still obscure [3] . Therefore, we knocked down Lck expression in OT-I primary CTLs using specific small hairpin RNA. After a decrease in Lck protein expression of about 60%, we were still able to observe CD3ζ phosphorylation to the same degree as control-treated cells after H2-K b -OVA tetramer stimulation ( Supplementary Figs 2 and 3a,e ). These data suggest either that Fyn is compensating for Lck absence, or that only a small pool of the total Lck is responsible for the initial phosphorylation. Free Lck is responsible for initial TCR–CD3 phosphorylation Our data strongly indicate that a free, rather than coreceptor-bound, pool of Lck initiates CD3 phosphorylation. To further investigate the role of free Lck in initiation of TCR signalling, we used Rag1 −/− OT-I mice in which Lck expression was controlled by the induction of a tetracycline-responsive transgene [41] . These mice are on an Lck −/− background, and induction of transgene expression with tetracycline successfully overcomes the lack of endogenous Lck, restoring normal thymopoiesis [41] . Withdrawal of the mice from tetracycline for at least 7 days (LckOFF) is sufficient to remove all residual protein [42] . We generated CTL from the LckOFF mice, and stimulated them with the agonist H-2K b -OVA tetramers. In this system, where there is no Lck present in the cells, there was no detectable phosphorylation of CD3ζ after specific OVA tetramer stimulation ( Fig. 7a ; Supplementary Fig. 3b ). CD3ζ phosphorylation was restored after transducing wild-type Lck into the Lck-deficient cells ( Fig. 7b , left; Supplementary Fig. 3c,d ). More interestingly, transducing the cells with a mutant version of the Lck protein that cannot interact with the coreceptor (C 20 A/C 23 A) [43] , restored substantial CD3ζ phosphorylation. To further investigate the contribution of free Lck to TCR antigen recognition at the immune synapse, we expressed wild-type or C 20 A/C 23 A mutant Lck fused to mCherry or eGFP, respectively, in LckOFF OT-I CTLs and monitored, using TIRFM, its localization during interactions with lipid bilayers presenting H2-K b -OVA and ICAM-1. Both wild-type (containing both free and coreceptor-bound forms) and mutant Lck pools were recruited to the immune synapse ( Fig. 8a ), strongly suggesting that Lck that is not associated with the CD8 coreceptor contributes to TCR signal initiation at the immune synapse. To differentiate the timing between coreceptor-associated Lck and free membrane-anchored Lck we prepared an OT-I T-cell hybridoma expressing CD3ζ-eGFP, a chimeric coreceptor formed by CD8α-Lck-Cerulean, CD8β-WT and a mutant Lck-C20.23A-mCherry (OT-I.ZG.8αLckC.8β.LckC2023A.R). We stimulated the cells using lipid bilayers containing H-2K b -OVA or H-2K b -VSV monomers and ICAM-1 for <1 min (early stimulation) or 2 min (late stimulation) and then performed colocalization analysis at the IS between free Lck and TCR, or coreceptor-associated Lck and TCR. The colocalization index when OVA was presented on the bilayer between free Lck and TCR was higher (0.72±0.02) at the earliest time point (0–30 s) than the index corresponding to coreceptor-associated Lck and TCR (0.54±0.01), whereas there were no significant differences between the indexes at 30–60 s (0.51±0.01 versus 0.50±0.01, respectively) or at any time point analysed when the bilayers contained VSV ( Fig. 8b ). These results strongly suggest that the free Lck initially interacts with TCR during antigen recognition, whereas coreceptor-bound Lck is recruited to the TCR/CD3 complex at later time points. 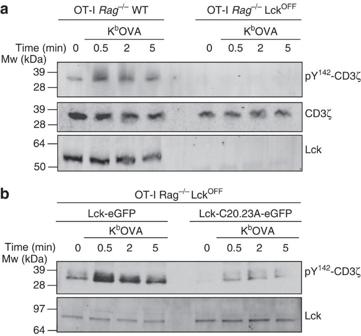Figure 7: Free Lck is responsible for initial TCR phosphorylation. (a) OT-IRag1−/−wild-type or LckOFFCTL were stimulated with H2-Kb-OVA tetramers for the indicated times. CD3ζ phosphorylation and Lck expression were analysed by immunoblot. Data are representative of three experiments. (b) OT-IRag1−/−LckOFFCTL cells were transduced with Lck-eGFP wild-type or with the mutant Lck(C20.23A)-eGFP and then stimulated with H2-Kb-OVA tetramers for the indicated times. CD3ζ phosphorylation and total Lck expression was analysed by immunoblot. Data are representative of two experiments. Figure 7: Free Lck is responsible for initial TCR phosphorylation. ( a ) OT-I Rag1 −/− wild-type or Lck OFF CTL were stimulated with H2-K b -OVA tetramers for the indicated times. CD3ζ phosphorylation and Lck expression were analysed by immunoblot. Data are representative of three experiments. ( b ) OT-I Rag1 −/− Lck OFF CTL cells were transduced with Lck-eGFP wild-type or with the mutant Lck(C20.23A)-eGFP and then stimulated with H2-K b -OVA tetramers for the indicated times. CD3ζ phosphorylation and total Lck expression was analysed by immunoblot. Data are representative of two experiments. 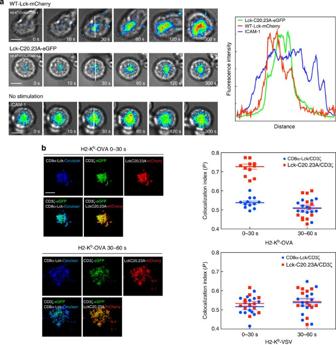Figure 8: Lck recruitment analysis. (a) OT-IRag1−/−CTL were transduced with wild-type mCherry-fused Lck (top row) or mutant Lck-C20.23A-eGFP (middle row), added to lipid bilayers containing H2-Kb-OVA monomers and ICAM-1(top two rows), or ICAM-1 only (bottom row), and the immune synapses were imaged under TIRF microscopy. Cells can be followed by transmitted light. Lck intensity is shown in false colour at selected time points. Scale bar, 5 μm. Bottom, intensity line profile of cells interacting with bilayers containing H2-Kb-OVA monomers and ICAM-1 (green) or ICAM-1 only (blue). Data are representative of three experiments. (b) Double colocalization analysis of immune synapses from OT-I.ZG.8αLckC.8β.Lck C2023A.R cells interacting with lipid bilayers containing H2-Kb-OVA (left) or H2-Kb-VSV(right) plus ICAM-1. Scale bar, 5 μm. Means±s.e.m. of two separate experiments of Pearson’s coefficient between CD3ζ-eGFP and Lck-C20.23A-mCherry (red squares) or CD3ζ-eGFP and CD8α-Lck-Cerulean (blue circles) were plotted. Full size image Figure 8: Lck recruitment analysis. ( a ) OT-I Rag1 −/− CTL were transduced with wild-type mCherry-fused Lck (top row) or mutant Lck-C20.23A-eGFP (middle row), added to lipid bilayers containing H2-K b -OVA monomers and ICAM-1(top two rows), or ICAM-1 only (bottom row), and the immune synapses were imaged under TIRF microscopy. Cells can be followed by transmitted light. Lck intensity is shown in false colour at selected time points. Scale bar, 5 μm. Bottom, intensity line profile of cells interacting with bilayers containing H2-K b -OVA monomers and ICAM-1 (green) or ICAM-1 only (blue). Data are representative of three experiments. ( b ) Double colocalization analysis of immune synapses from OT-I.ZG.8αLckC.8β.Lck C2023A.R cells interacting with lipid bilayers containing H2-K b -OVA (left) or H2-K b -VSV(right) plus ICAM-1. Scale bar, 5 μm. Means±s.e.m. of two separate experiments of Pearson’s coefficient between CD3ζ-eGFP and Lck-C20.23A-mCherry (red squares) or CD3ζ-eGFP and CD8α-Lck-Cerulean (blue circles) were plotted. Full size image Early T-cell signalling events such as LAT phosphorylation or calcium flux take place within a few seconds [8] . Performing higher-spatial/temporal resolution experiments using a supported lipid bilayer system as a surrogate antigen-presenting surface, we have been able to image TCR–CD8 FRET in small regions within the IS. These were too localized to show a signal above the background when FRET signals were averaged over the whole synapse, explaining why they were not noticed before in regular live or fixed epifluorescence experiments [24] . A recent study on TCR and CD8 binding to MHCp showed that there is a two-stage interaction process in which first TCR interacts with MHCp and, after an SFK-mediated activity, there is a stabilization phase carried out by CD8–MHCp binding [3] , [9] . This was identified using blocking antibodies against CD8 and the SFK inhibitor PP2, where only the first phase of the interaction takes place [9] . Our new FRET/TIRF data show a small but significant increase in FRET signal within 1 min of adding cells to the imaging chamber, followed by a second, stronger, increase after about 5 min. This suggests that the early FRET signal represents CD8 brought passively to the TCR by binding of Lck to phospho-CD3 or phospho-ZAP70. The later, stronger FRET was likely due to stabilization of the TCR–MHCp complex by CD8 binding to MHCI, because of the absence of induction of the FRET signal or Tyr-phosphorylation in cells expressing a mutant CD8 that cannot bind MHCI. This suggested that the interaction operative at early stages goes away over time. Moreover, when cells expressed a CD8 mutant that cannot bind Lck, there was only a low FRET signal, demonstrating that the Lck interaction with CD8 was required to bring CD8 close to the TCR. It might be possible that the interaction between MHCI and CD8 is strong enough to overcome this effect at later time points, as suggested by the recovery of the second interaction stage. These results were supported using the same biophysics approach conducted by Jiang et al. [9] in their work. Using OT-I T-cell hybridomas we were able to detect a two-stage interaction kinetic between TCR–CD8 and MHCp only when cells expressed wild-type CD8 molecules. When the cells expressed either the Lck–CD8-binding mutant or MHC–CD8-binding mutant, only the first stage of the interaction was detectable. It is commonly accepted that CD8 is recruited to the signalling TCR by its MHCp interaction. However, if the CD8–MHCp interaction does not happen until after TCR ITAMs are phosphorylated, how is the initial CD8 recruitment produced? One possibility supported by our data is that passive diffusion would allow Lck to bind to the phosphorylated ITAMs on the TCR, or even directly to phospho-ZAP70, thus bringing any coreceptor-associated Lck passively to the TCR. An earlier study with chimeras of CD4–Lck showed that mutation of the Lck SH2 domain in the chimera reduced the ability to restore thymopoiesis independently of the kinase activity, suggesting a protein–protein interaction role for Lck [18] . Although Lck phosphorylation of TCR ITAMs is one of the earliest detected events in T-cell activation, it still remains unsolved. Briefly, Lck activity is controlled by a balance between phosphorylation of two main tyrosine residues, Tyr 394 , known to promote an open active conformation, and Tyr 505 , known to promote a closed inactive conformation [12] , [44] . Conflicting data on this subject are available. Most traditional biochemical studies showed no changes on the phosphorylation level of Lck after TCR stimulation, so Lck could be accessible to very subtle regulatory mechanisms without the need for acute changes in Tyr 505 and Tyr 394 phosphorylation and conformational alterations, as FRET studies with an Lck sensor claimed [45] . On the other hand, more fine measurements with the same sensor, analysing its fluorescence lifetime, enabled the direct visualization of the dynamic local opening of 20% of the total amount of Lck proteins after activation of T cells with Ab against CD3, or by superantigen-loaded APCs [46] . Nika et al. [15] reported that up to 40% of total Lck present in unstimulated naive T cells and thymocytes was constitutively active, consistent with the data obtained with the fluorescent Lck reporter construct [45] , [46] . This substantial, pre-existing pool of active Lck molecules in the membrane of resting T cells might be sufficient to mediate phosphorylation of the TCR. To address this question, we have found that a mutant Lck (C 20 A/C 23 A) that cannot bind to CD8 was able to restore induction of TCR phosphorylation and showed a higher colocalization index with TCR after MHCp recognition than did coreceptor-associated Lck. This was similar to the effect of wild-type Lck in Lck-deficient cells after T-cell stimulation. Given these findings, we propose a model in which before TCR interaction with MHCp, some Lck is associated with the plasma membrane, with some Lck also associated with CD8. Upon TCR binding to MHCp, non-CD8-bound Lck becomes associated with the TCR–CD3 complex, and phosphorylates CD3ζ ITAMs and then ZAP70, which binds to the phosphorylated CD3ζ ITAMs. The SH2 domain of CD8-bound Lck then interacts with phospho-ZAP70, pulling CD8 into proximity with the MHCp-interacting TCR [47] , [48] . The extracellular immunoglobulin domains then bind to the MHCp, stabilizing the TCR–MHCp interaction. Mice B6 mice were bred at NUS. All experimental procedures performed in Singapore were approved by the institutional animal care and use committees of the National University of Singapore. OT-I, OT-I Rag1 −/− mice all on the B6 background were bred at The Scripps Research Institute and were maintained in accordance with the Animal Care and Use Committee of The Scripps Research Institute. OT-I Rag1 −/− Lck OFF spleens were provided by Rose Zamoyska (School of Biological Sciences, University of Edinburgh). Mice of either sex were used between 5 and 8 weeks of age. Mice were age and sex matched in each experiment. Constructs and cells CHO cells expressing the tetracycline repressor (Invitrogen TRex) under blasticidin selection (10 μg ml −1 ) were grown in Ham’s F12 media with 10% (vol/vol) FCS, 100 U ml −1 of penicillin, 10 mg ml −1 of streptomycin, hygromycin 0.3 mg ml −1 and G418 0.8 mg ml −1 . CTLs were prepared from OT-I transgenic mouse spleen cell suspensions. RBCs were lysed with ACK buffer, and the cell suspension was cultured in an upright T75 flask, in complete RPMI (10% fetal bovine serum, 50 mM β-ME, 2 mM L-glutamine, 100 U ml −1 penicillin and 10 mg ml −1 streptomycin) plus 10 U ml −1 IL-2 plus 10 nM OVA peptide for 48–72 h. The cells were washed to remove peptide and resuspended in fresh medium with IL-2. CTLs were used from day-5 cultures. For continued culture, after 7–10 days culture and expansion in the presence of IL-2, CD8 + cells were restimulated at 7–10-day intervals. Cells (1 × 10 6 per ml) were restimulated with 3 × 10 6 irradiated (3,000 rads) B6 spleen cells previously pulsed with 5 μg ml −1 OVA for 30 min. Hybridomas expressing the OT-I TCR with or without CD8α and CD8β were made by retroviral transfection of TCR-deficient 58α−β− cells [49] . Chimeric genes encoding CD8β-YFP, CD8β-mCherry, CD3ζ-CFP [21] , CD3ζ-eGFP, and Lck-eGFP, Lck-mCherry and CD8α-Lck-Cerulean were constructed, inserted into retroviral vector pBMN-Z (S. Kinoshita and G. Nolan, www.stanford.edu/group/nolan ) and were expressed in Plat-E packaging cells. All the mutants were made using the Quickchange Site Mutagenesis Kit (Stratagene). Supernatants of these cells were used to transduce OT-I hybridomas and OT-I CTL. For optimal FRET sensitivity and to avoid false-negative results, the acceptor (YFP or mCherry) should be in excess relative to the donor (CFP or eGFP). Clones were selected based on the optimal acceptor/donor molar ratio for FRET; that is, an acceptor/donor molar ratio of 1:1 to 3:1. mCherry-tSH2(ZAP70) [36] (Addgene plasmid 27137) was cloned into pBMN-Z vector using Hind-III and Not-I sites. Two different sequences were used for Lck knockdown in pGFP-RS-U6 small hairpin RNA vector (#232#ctgcaagacaacctggtta and #43# gagaacattgacgtgtgtg). OT-I hybridoma cells were maintained in IMDM medium containing 10% fetal bovine serum, 2 mM L-glutamine, 100 U ml −1 penicillin/streptomycin, 50 mM β-mercaptoethanol, 500 μg ml −1 G418 (selecting for TCRα) and 3 μg ml −1 puromycin (selecting for TCRβ). FRET microscopy A dual-camera system specifically designed for FRET imaging was used for imaging, allowing simultaneous acquisition of donor emission and acceptor emission during donor excitation and fast changes between donor and acceptor excitation. This consisted of two CoolSnapHQ cameras (Roper) attached to a Zeiss 200M microscope through a beam splitter (custom 520LPXR; Chroma) and stationary emission filters. A DG4 galvo illuminator customized with a 300-W xenon lamp (Sutter) was used for rapid wavelength switching. The system was run by Slidebook 6.0 software (3I). The optical filters were as follows (center/bandpass): YFP excitation, 504/12–25 nm; YFP emission, 542/27 nm; CFP excitation, 427/10 nm; CFP emission, 472/30 nm; mCherry excitation, 589/15 nm; mCherry emission, 632/22 nm; Cy5 excitation, 620/52 nm; Cy5 emission, 675/50 nm. Beamsplitting was achieved with a dichroic mirror (Chroma). Exposure times were 0.2–0.5 s, with 2 × 2 binning and a × 100, 1.4 numerical aperture oil objective, and software flatfield correction was used. Live cells were imaged in Hank’s balanced salt solution (HBSS) medium supplemented with 1 mM CaCl 2 , 1 mM MgCl 2 and 10 mM HEPES and without antibiotics and were maintained at 37 °C by the FCS2 live-imaging chamber and objective heater (Bioptechs). APCs were added to a prewarmed imaging chamber coated with poly- D -lysine (Sigma). For fixed-cell imaging, cells were mounted in Slowfade Light antifade mounting media (Molecular Probes). TIRF microscopy TIRF microscopy experiments were performed using a × 100 1.45 numerical aperture TIRF objective (Nikon) on a Nikon TE2000U microscope custom modified with a TIRF illumination module. Laser illumination (488 and 561 nm laser lines) were adjusted to impinge on the coverslip at an angle to yield a calculated evanescent field depth ( d ) <100 nm. Images were acquired on a 14 bit, cooled charge-coupled device camera (CoolSnap HQ [2] , Roper) controlled through NIS-Elements software (Nikon Inc.). The images were recorded using 300–500-ms exposures depending on the fluorescence intensity of the sample. In some experiments an Olympus IX83 inverted microscope equipped with a four-laser (405, 488, 561 and 647 nm) motorized TIRF module was used and images were obtained in a Hamamatsu ORCA Flash 4.0 camera. FRET analysis Crosstalk compensation and extraction of donor-normalized FRET was performed using a three-filter set algorithm as described previously [21] , [30] , [50] . For each focal position, three exposures were registered: I DD (donor excitation/donor emission), I AA (acceptor excitation/acceptor) and I DA (donor excitation/acceptor, or more generally DA). Background was subtracted based on local fluorescence averaged from a user-specified, cell-free region of each image. The bleed-through coefficients of donor into the DA image and acceptor into the DA image were calibrated using T cells transfected with either CD3ζ-donor or CD8β-acceptor alone. Acceptor>DA bleed-through was a =12% for eYFP in the dual-camera system and a =7.5% for mCherry in the TIRF system, donor>DA bleed-through was d =54% for eCFP in the dual-camera system and d =10.6% for eGFP in the TIRF system. Sensitized emission was calculated by simply correcting the DA image for donor and acceptor bleed-through: F c = I DA −a* I AA −d* I DD . To get FRET efficiency ( E ), we used the following formula: E app = F c /( F c +( G * I DD )), where G is the independently calibrated ratio of sensitized emission in the I DA filter set before photobleaching, to donor recovery in the I DD filter set after acceptor photobleaching. For eCFP and eYFP in the dual-camera system G =3.83±0.1, for eGFP and mCherry in the TIRF system G =2.1±0.1. We have implemented this FRET method as an available upon request ImageJ plugin modified from Roszik et al. [51] The FRET image was masked to accept only regions in which donor intensity was >4 times above background noise. Cells with donor/acceptor ratios outside the stoichiometric range of 1:1 to 3:1, as well as movement artefacts, were excluded from analysis. The average FRET was calculated from the synapse. Ca 2+ flux imaging H2-K b -OVA-expressing CHO cells were plated in poly- D -lysine-coated chambers then, after washing in Ca 2+ /Mg 2+ -free medium containing 1 mM EGTA, OT-I T-cell hybridoma cells expressing both CD8α and CD8β loaded with 2 μM Ca 2+ -sensitive dye Fluo-4 were added on top. Imaging of Fluo-4 fluorescence was conducted in HBSS supplemented with 2.5 mM CaCl 2 , 2.5 mM MgCl 2 and 10 mM HEPES. In the case of primary cells, Fluo-4-loaded CTLs were added to lipid bilayers containing the apropiate antigen, after allowing cells to settle in Ca 2+ /Mg 2+ -free medium containing 1 mM EGTA, one volume of prewarmed HBSS supplemented with 2.5 mM CaCl 2 , 2.5 mM MgCl 2 and 10 mM HEPES was added. Cell surface molecular density and Adhesion Frequency Assay For every micropipette experiment, site densities of MHCp on RBCs and TCR and CD8 on T cells were measured by flow cytometry. To measure the MHCp site density, RBCs were incubated with PE-conjugated monoclonal Ab 3H2672 (for H-2K b ) at 10 μg ml −1 in 200 μl of FACS buffer (RPMI 1640, 5 mM EDTA, 1% BSA and 0.02% sodium azide) on ice for 40 min. Similarly, CD8α subunit (clone 53-6.7), CD8β subunit (clone H35-17.2), TCR Vα2 (clone B20.1) and CD3ε (clone 145-2-C11) expressed on T cells were stained with their respective PE-conjugated monoclonal Abs (1:300 dilution, eBiosciences). CD8 is expressed as either an αα homodimer or an αβ heterodimer. Therefore, it is assumed that the site density of CD8αβ equals that of CD8β, whereas the site density of CD8αα equals half of the site-density difference between CD8α and CD8β. For the adhesion frequency assay [35] , an OT-I T cell and a RBC were aspirated by respective pipettes and driven in and out of contact with controlled area and duration. Adhesion was observed from stretching of the RBC on T-cell retraction. This contact–retraction cycle was either repeated 50 times for a given contact duration on each cell pair, and 3–5 cell pairs were used to estimate an adhesion frequency P a (mean±s.e.m.). P a can be converted to the average number <n> by < n >=1−ln(1− P a ) and divided by ligand density m pMHC to obtain normalized adhesion bonds <n>/m pMHC . Experiments were performed at room temperature. Liposomes and lipid bilayer preparation 1,2-dioleoyl-sn-glycero-3-phosphocholine was mixed in chloroform with 0.2 mol% 1,2-dioleoyl-sn-glycero-3-[( N -(5-amino-1-carboxypentyl) iminodiacetic acid)succinyl] (Ni-NTA-DOGS) and 0.2 mol% 1,2-dioleoyl-sn-glycero-3-phosphoethanolamine- N -Cap-Biotinyl (CAP-biotin-PE), all the lipids were from Avanti Polar Lipids, dried under vacuum and sonicated in 2% OG. The liposome solution was then extruded through a 0.22-μm filter and dialysed against 4 l of Tris saline buffer (Tris-HCl 20 mM, NaCl 50 mM). Glass slides (No. 1, 24 mm × 50 mm German borosilicate; Menzel-Gläser) were treated with Piranha solution (70% sulfuric acid and 30% hydrogen peroxide) (both from Sigma-Aldrich) for 20 min, rinsed with doubly distilled or deionized water, dried in air and attached with epoxy glue to the bottom of 8-well LabTek II chambers (Nunc), from which the glass bottom had been removed. Slides were exposed to a 10-fold-diluted lipid suspension for 10 min and rinsed with HEPES–Na buffer (150 mM NaCl, 5 mM HEPES (pH 7.4)). NiSO 4 (0.25 mM) was introduced into the chamber for 10 min to charge NTA-DOGS with Ni 2+ . Lipid bilayers were then blocked with blocking buffer (5 mg ml −1 BSA in HEPES–Na buffer (pH 7.4)) in the presence of 1 μg ml −1 His-tagged ICAM-1 for 30 min. The blocked bilayer was incubated sequentially with 1 μg ml −1 streptavidin for 30 min followed by 1 μg ml −1 H2-K b -peptide for 1 h. After washing, the bilayers were imaged in HBSS supplemented with 1 mM CaCl 2 , 1 mM MgCl 2 and 10 mM HEPES. Immunoblots Cells (5 × 10 6 ) were lysed in 1% Brij96, 50 mM HEPES, pH 7.4, 150 mM NaCl, 1 mM Na 3 VO 4 , 1 mM phenylmethyl sulphonyl fluoride and a protease inhibitor ‘cocktail’, and the cell lysates were separated by 10% reducing SDS–polyacrylamide gel electrophoresis, and transferred to PVDF membrane. The membranes were incubated with specific primary antibodies followed by incubation with goat anti-rabbit IgG (H1L), DyLight 800-conjugated (Pierce, #35571) or goat anti-mouse IgG (H1L), DyLight 680-conjugated (Pierce, #35519) and detected and quantified with a LiCor Odyssey infrared imaging system. Colocalization analysis This was performed with JACoP plugin in ImageJ. Background levels were obtained by measuring the mean intensity of each signal outside the cells and were subtracted; negative pixel values were clipped to zero. Pearson’s P colocalization index was calculated. How to cite this article: Casas, J. et al. Ligand-engaged TCR is triggered by Lck not associated with CD8 coreceptor. Nat. Commun. 5:5624 doi: 10.1038/ncomms6624 (2014).